A phosphatidylinositol-4-phosphate powered exchange mechanism to create a lipid gradient between membranes Lipids are unevenly distributed within eukaryotic cells, thus defining organelle identity. How non-vesicular transport mechanisms generate these lipid gradients between membranes remains a central question. Here using quantitative, real-time lipid transport assays, we demonstrate that Osh4p, a sterol/phosphatidylinositol-4-phosphate (PI(4)P) exchanger of the ORP/Osh family, transports sterol against its gradient between two membranes by dissipating the energy of a PI(4)P gradient. Sterol transport is sustained through the maintenance of this PI(4)P gradient by the PI(4)P-phosphatase Sac1p. Differences in lipid packing between membranes can stabilize sterol gradients generated by Osh4p and modulate its lipid exchange capacity. The ability of Osh4p to recognize sterol and PI(4)P via distinct modalities and the dynamics of its N-terminal lid govern its activity. We thus demonstrate that an intracellular lipid transfer protein actively functions to create a lipid gradient between membranes. Sterol is a key lipid in eukaryotic cells that, owing to its rigid and planar structure, reduces the flexibility of neighbouring lipids, thereby ensuring the impermeability of membranes [1] . The endoplasmic reticulum (ER), in which sterol is synthesized, displays low sterol levels (<5 mol% of lipids) [2] . Contrastingly, sterol is abundant (up to 40 mol%) in the trans -Golgi, endosomes and plasma membrane (PM) [3] , [4] . This gradient between early and late regions of the secretory pathway is supposed to be mainly established by specialized lipid transfer proteins (LTPs) [5] , [6] able to transport sterol, insoluble in aqueous media, between membranes [7] , [8] . Some LTPs for sterol belong to the oxysterol-binding protein-related proteins (ORP)/Osh family, an evolutionary conserved family in eukaryotes, including ORP in human and oxysterol-binding homologue (Osh) proteins in yeast [9] . In higher eukaryotes, members of the START family are also potential LTPs for sterol [10] . Defining the mechanisms by which LTPs create intracellular sterol gradients remains a central issue in membrane biology [7] , [8] . One model posits that LTPs randomly equilibrate sterol between subcellular membranes by bidirectional shuttling [5] , [11] . The accumulation of sterol in the trans -Golgi and PM would be merely driven by its high affinity for saturated glycerophospholipids and sphingolipids [12] , [13] , [14] , largely abundant in these compartments [3] , [15] , [16] . An alternative hypothesis, suggested by our recent studies on ORP/Osh proteins, is that LTPs actively create sterol gradients by vectorial transport [17] , [18] . Osh4p is an archetypical LTP whose structure consists of a 19-strand β-barrel defining a sterol-binding pocket [19] . A short N-terminal segment forms a lid that blocks the sterol molecule inside its binding cavity. We revealed that Osh4p can alternatively extract PI(4)P from a membrane. X-ray crystallography indicated that the sterol-binding pocket accommodates the PI(4)P acyl chains, whereas charged residues defining an adjacent pocket recognize the PI(4)P headgroup. The lid, under a different conformation, shields the lipid. Strikingly, we observed that Osh4p transfers sterol and PI(4)P along opposed directions between membranes by counterexchange [17] . PI(4)P is mostly localized in the trans -Golgi and PM [20] but is absent from the ER, implying that a steep PI(4)P gradient exists between these distinct cellular regions. In yeast this gradient is maintained by spatially distant enzymes. Pik1p and Stt4p phosphorylate PI into PI(4)P in the trans -Golgi and PM, respectively [20] , whereas Sac1p, the major phosphatase that degrades PI(4)P into PI [21] , [22] , resides at the ER [23] . Intriguingly, Osh4p downregulates cellular PI(4)P levels and the availability of this lipid on Golgi surface, thereby counteracting Pik1p and Sec14p [24] , a PI/PC LTP that teams with Pik1p to yield Golgi PI(4)P [25] . Several reports also suggest that Osh4p supplies the trans -Golgi and PM with sterol [26] , [27] , [28] . Consequently, we proposed that Osh4p uses the PI(4)P gradient at the ER/Golgi interface to supply the trans -Golgi with sterol. In our model, Osh4p extracts sterol from the ER, then releases it by counter exchange with PI(4)P at the Golgi, and transports PI(4)P from the Golgi to the ER. The ATP-dependant production of PI(4)P by Pik1p would energetically drive sterol/PI(4)P cycles by Osh4p, thereby promoting the active release of sterol into the trans- Golgi and the creation of a sterol gradient ( Fig. 1 ). 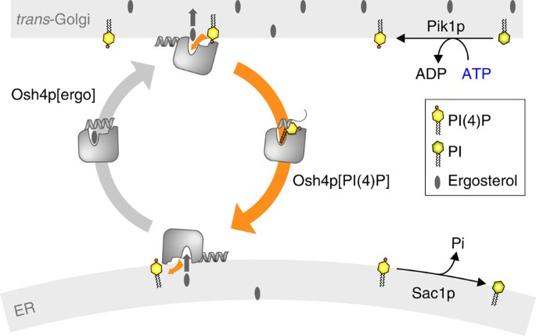Figure 1: Working model of sterol/PI(4)P transport cycles mediated by Osh4p at the ER/Golgi interface. Osh4p would transport ergosterol from the ER to the trans-Golgi and PI(4)P in the reverse direction by sterol/PI(4)P exchange. ATP-dependent phosphorylation of PI into PI(4)P by Pik1p and hydrolysis of PI(4)P by Sac1p would fuel multiple sterol/PI(4)P exchange cycles and, thereby, the creation and maintenance of a sterol gradient. Figure 1: Working model of sterol/PI(4)P transport cycles mediated by Osh4p at the ER/Golgi interface. Osh4p would transport ergosterol from the ER to the trans-Golgi and PI(4)P in the reverse direction by sterol/PI(4)P exchange. ATP-dependent phosphorylation of PI into PI(4)P by Pik1p and hydrolysis of PI(4)P by Sac1p would fuel multiple sterol/PI(4)P exchange cycles and, thereby, the creation and maintenance of a sterol gradient. Full size image Here we have tested this model using novel quantitative and real-time assays to measure the transfer of sterol and PI(4)P between liposomes mimicking the ER/Golgi interface. We demonstrate that Osh4p transports sterol at high velocity and, remarkably, even against a sterol concentration gradient, by dissipating a PI(4)P gradient. The maintenance of this PI(4)P gradient over time sustains sterol transport by Osh4p. Differences in lipid packing between membranes influence the transfer of lipids and stabilize sterol gradients created by Osh4p. Its activity relies on the dynamic of its N-terminal lid. Our results provide the first demonstration that an intracellular LTP has a built-in capacity to actively create a lipid gradient between membranes. Osh4p mediates fast sterol/PI(4)P exchange To measure the sterol/PI(4)P exchange capacity of Osh4p, we devised two fluorescence resonance energy transfer (FRET)-based assays with high temporal resolution to quantify sterol transport from ER- to Golgi-like liposomes (L E and L G liposome, Fig. 2a ) and PI(4)P transport in the backward direction ( Fig. 2b ). 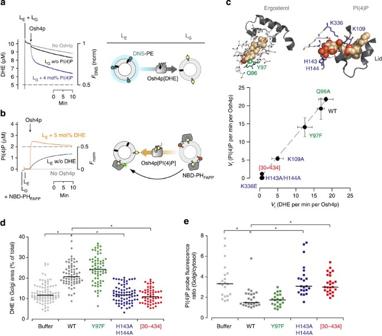Figure 2: Coupling of DHE and PI(4)P transport by Osh4p between ER- and Golgi-like liposomes. (a) DHE transport assay. DOPC/DNS-PE/DHE liposomes (92.5/2.5/5 mol/mol, 200 μM total lipids, LE) were mixed with DOPC liposomes (200 μM lipids, LG) containing, or not, 4 mol% PI(4)P at 30 °C. After 3 min, Osh4p (200 nM) was added. FRET between DHE and DNS-PE in the LEliposomes diminishes as DHE is transported to the LGliposomes. The signal was converted into amount of DHE present in LEliposome (in μM). The slow decay observed without Osh4p was due to spontaneous DHE transfer. The dashed line corresponds to full equilibration of DHE between liposomes. (b) PI(4)P transport assay. DOPC/PI(4)P/Rhod-PE liposomes (94/4/2 mol/mol, 200 μM lipids, LG) were incubated with NBD-PHFAPP(250 nM). Then DOPC liposomes (200 μM lipids, LE) containing, or not, 5 mol% DHE were added. After 3 min, Osh4p (200 nM) was injected. The dequenching of NBD signal mirrors the translocation of NBD-PHFAPPfrom LGto LEliposomes. The dashed line corresponds to the signal of NBD-PHFAPPobtained under conditions mimicking full PI(4)P equilibration between liposomes. (c) Plot of initial DHE transport rates versus initial PI(4)P transport rates for Osh4p WT or mutants (200 nM) measured with LEand LGliposomes containing 5 mol% DHE and 4 mol% PI(4)P, respectively. Data are represented as mean±s.e.m. (horizontal and vertical error bars,n=2). Localization of key residues (in stick with nitrogen in blue, and oxygen in red) are shown in a close-up view of the PI(4)P headgroup or sterol-binding pocket. The H-bonds are represented. (d) Osh4p or mutants were microinjected into HeLa cells doped with DHE. The plot shows the amount of DHE in the Golgi area (n=50–90 cells for each condition; *P<0.001 (Student’st-test). (e) Osh4p or mutants were microinjected into HeLa cells expressing the GFP-tagged PHOSBPprobe. The plot shows the ratio of PI(4)P probe in the Golgi versus cytosol areas (n=20–25 cells; *P<0.001). Figure 2: Coupling of DHE and PI(4)P transport by Osh4p between ER- and Golgi-like liposomes. ( a ) DHE transport assay. DOPC/DNS-PE/DHE liposomes (92.5/2.5/5 mol/mol, 200 μM total lipids, L E ) were mixed with DOPC liposomes (200 μM lipids, L G ) containing, or not, 4 mol% PI(4)P at 30 °C. After 3 min, Osh4p (200 nM) was added. FRET between DHE and DNS-PE in the L E liposomes diminishes as DHE is transported to the L G liposomes. The signal was converted into amount of DHE present in L E liposome (in μM). The slow decay observed without Osh4p was due to spontaneous DHE transfer. The dashed line corresponds to full equilibration of DHE between liposomes. ( b ) PI(4)P transport assay. DOPC/PI(4)P/Rhod-PE liposomes (94/4/2 mol/mol, 200 μM lipids, L G ) were incubated with NBD-PH FAPP (250 nM). Then DOPC liposomes (200 μM lipids, L E ) containing, or not, 5 mol% DHE were added. After 3 min, Osh4p (200 nM) was injected. The dequenching of NBD signal mirrors the translocation of NBD-PH FAPP from L G to L E liposomes. The dashed line corresponds to the signal of NBD-PH FAPP obtained under conditions mimicking full PI(4)P equilibration between liposomes. ( c ) Plot of initial DHE transport rates versus initial PI(4)P transport rates for Osh4p WT or mutants (200 nM) measured with L E and L G liposomes containing 5 mol% DHE and 4 mol% PI(4)P, respectively. Data are represented as mean±s.e.m. (horizontal and vertical error bars, n =2). Localization of key residues (in stick with nitrogen in blue, and oxygen in red) are shown in a close-up view of the PI(4)P headgroup or sterol-binding pocket. The H-bonds are represented. ( d ) Osh4p or mutants were microinjected into HeLa cells doped with DHE. The plot shows the amount of DHE in the Golgi area ( n =50–90 cells for each condition; * P <0.001 (Student’s t -test). ( e ) Osh4p or mutants were microinjected into HeLa cells expressing the GFP-tagged PH OSBP probe. The plot shows the ratio of PI(4)P probe in the Golgi versus cytosol areas ( n =20–25 cells; * P <0.001). Full size image In the first assay, L E liposomes contained both dehydroergosterol (DHE, 5 mol%) and 1,2-dioleoyl-sn-glycero-3-phosphoethanolamine-N-(5-dimethylamino-1-naphthalenesulfonyl) (DNS-PE, 2.5 mol%), whereas L G liposomes incorporated, or not, 4 mol% PI(4)P. The decrease in FRET between DHE and DNS-PE allows quantifying the transport of DHE by Osh4p (200 nM) from L E to L G liposomes [17] . When L G liposomes were devoid of PI(4)P, the initial DHE transport rate was slow ( Fig. 2a , black trace, 1±0.1 DHE per min per protein (mean±s.e.m., n =4)). Contrastingly, when L G liposomes contained PI(4)P, the transport rate was 17 times higher ( Fig. 2a , blue trace, 17.4±1.1 DHE per min per protein ( n =6)). The efficacy of Osh4p to transport DHE was directly proportional to PI(4)P amounts initially present in L G liposomes ( Supplementary Fig. 1 ). These results corroborated our previous observations [17] . To measure the back transport of PI(4)P from L G to L E liposomes, we created a PI(4)P sensor based on the FAPP1 PH domain (PH FAPP ). This domain has a binding site for the PI(4)P headgroup and a hydrophobic wedge that inserts into membranes [29] . We produced a PH FAPP domain including a single solvent-exposed cysteine (C13), localized in the hydrophobic wedge, to which we grafted a polarity-sensitive NBD (7-nitrobenz-2-oxa-1,3-diazol) probe ( Supplementary Fig. 2a–c ). Incremental addition of liposomes doped with 2 mol% PI(4)P to the NBD-PH FAPP construct resulted in a blue shift of the maximal emission wavelength of NBD from 542 to 529 nm with a maximal sixfold increase in intensity ( Supplementary Fig. 2d,e ). A similar binding curve was obtained with liposomes containing PI(4)P and high DHE levels (10 mol%). No binding was seen with liposomes devoid of PI(4)P or containing 2 mol% PI. Thus, NBD-PH FAPP is a specific sensor of PI(4)P and its response is independent of sterol levels. In the transport assay ( Fig. 2b ), NBD-PH FAPP (250 nM) was mixed with L G liposomes doped with 4 mol% PI(4)P and 2 mol% Rhod-PE (1,2-dipalmitoyl- sn -glycero-3-phosphoethanolamine-N-(lissamine rhodamine B sulfonyl)). The NBD fluorescence was quenched due to a FRET process with Rhod-PE. Adding L E liposomes did not induce any signal increase: all NBD-PH FAPP copies remained associated with L G liposomes. The subsequent injection of Osh4p (200 nM) provoked a fast dequenching, indicative of the transport of PI(4)P by Osh4p and translocation of NBD-PH FAPP to L E liposomes ( Fig. 2b ). To quantify this transport, the NBD signal was normalized (see Methods) by taking as reference the NBD signal measured in a condition mimicking full PI(4)P equilibration between L E and L G liposomes, each containing 2 mol% PI(4)P ( Supplementary Fig. 2f ). With DHE-free L E liposomes, Osh4p transported PI(4)P with an initial rate of 1.9±0.6 PI(4)P per min ( n =3) ( Fig. 2b , black trace). Strikingly, with L E liposomes containing 5 mol% DHE, the transport rate was accelerated by 1 order of magnitude (22.2±0.7 PI(4)P per min per protein ( n =8)) resulting in PI(4)P equilibration between the two liposome populations within 1 min ( Fig. 2b , orange trace). Remarkably, the initial PI(4)P transport rate was similar to that measured for DHE under the same condition, DHE and PI(4)P being present in distinct membranes. This correlation between lipid transport velocities as measured along opposite directions strongly indicated that Osh4p is a sterol/PI(4)P exchanger. Sterol/PI(4)P exchange activity of Osh4p mutants To further address the coupling between sterol and PI(4)P transport, we tested mutants lacking residues that make major contact with either sterol (Q96A and Y97F) [19] or PI(4)P (K109A, K336E and H143A/H144A) [17] . If the transport of the two lipids relies on a counter-exchange mechanism, then affecting the binding of one lipid ligand should affect the transport of the second ligand. We first assessed the ability of Osh4p mutants to extract lipids. Surprisingly, the Q96A and Y97F mutants were not deficient in extracting DHE ( Supplementary Fig. 3a ). Mutants belonging to the second group (K109A, K336E and H143A/H144A) properly extracted DHE [17] but not PI(4)P ( Supplementary Fig. 3b ). Like Osh4p wild type (WT), all mutants slowly transported DHE or PI(4)P between membranes in the absence of the second lipid ( Supplementary Fig. 3c ). However, in transport assays including both lipids, the K336E and H143A/H144A mutants displayed no sterol/PI(4)P exchange activity compared with Osh4p WT, whereas the K109A mutant retained some residual activity, as indicated by both the initial DHE and PI(4)P transport velocities ( Fig. 2c , Supplementary Fig. 3c ). The Y97F mutant (but not the Q96A mutant) was slightly less active than Osh4p WT. Finally, we found that the lidless [30–434]Osh4p mutant was unable to properly extract PI(4)P or DHE and to exchange lipids, indicating that the lid is a key structural element for the function of Osh4p ( Supplementary Fig. 3a–c , Fig. 2c ). This structure-function analysis shows that the sterol and PI(4)P transport processes are intimately coupled and occur efficiently only when Osh4p properly recognizes the two lipids. This confirms that Osh4p is a sterol/PI(4)P exchanger. Next, we tested whether Osh4p WT can displace sterol and PI(4)P in a cellular context. First, we microinjected recombinant Osh4p WT into HeLa cells supplied with DHE. Remarkably, Osh4p WT promoted an enrichment of the Golgi area with DHE compared with experiments in which only buffer was injected ( Fig. 2d , Supplementary Fig. 4a,b ). Immunostaining of the cells with anti-TGN46 antibody indicated that DHE was mostly localized in the trans -Golgi ( Supplementary Fig. 4a ). Next, we microinjected Osh4p in cells expressing the PI(4)P-specific probe green fluorescent protein (GFP)-tagged PH OSBP . In control cells, the probe was localized at the Golgi, whereas in the presence of Osh4p the probe was mostly cytosolic, indicating that PI(4)P Golgi levels were lowered ( Fig. 2e , Supplementary Fig. 4c ). Last, we repeated the experiments with Osh4p mutants. The Y97F mutant had the same activity as Osh4p WT ( Fig. 2d,e , Supplementary Fig. 4b,c ). Contrastingly, the H143A/H144A and [30–434] mutants failed to deliver DHE to the Golgi region and to displace PI(4)P. Altogether, these cellular observations match perfectly the in vitro results and indicate that Osh4p must recognize and displace PI(4)P from the Golgi to supply it with sterol, thereby corroborating our model on its sterol/PI(4)P exchange function. Maintaining a PI(4)P gradient sustains sterol transfer The DHE transport kinetic measured in the presence of PI(4)P was biphasic ( Fig. 2a ). The first phase corresponds to the sterol/PI(4)P exchange and ends when PI(4)P is equilibrated between liposomes. A similar amount of DHE and PI(4)P is exchanged ( ∼ 2 μM, Fig. 2a,b ). The second phase likely corresponds to the slow completion of DHE equilibration by Osh4p since, in our assays, the amount of DHE to be transported is higher than the amount of PI(4)P. Thus Osh4p efficiently transports DHE, by sterol/PI(4)P exchange, from ER to Golgi-like membranes until it has fully equilibrated the PI(4)P gradient, which pre-existed between these membranes. In yeast, PI(4)P gradients between the ER and late membranes are maintained by PI4-kinases and Sac1p [21] , [23] . This might sustain sterol/PI(4)P exchange cycles by Osh4p. To examine this hypothesis in vitro , we attached a Sac1p[1–522]His 6 construct (200 nM), in which the His-tag substitutes for the TM region, to L E liposomes doped with DOGS-NTA-Ni 2+ (1,2-dioleoyl- sn -glycero-3-[(N-(5-amino-1-carboxypentyl)iminodiacetic acid)succinyl]). Flotation assays indicated that Sac1p[1–522]His 6 was fully and selectively attached to such liposomes ( Supplementary Fig. 5a ). With Sac1p bound to L E liposomes and under conditions where L G liposomes included PI(4)P, the biphasic aspect of the DHE transport kinetics mediated by Osh4p was lost ( Fig. 3a , cyan trace). The transport of DHE was sustained over time and, at the end of the kinetic more DHE (1 μM) was transferred into L G liposomes compared with the experiment without Sac1p. This effect is due to the hydrolysis of PI(4)P: an inactive Sac1p mutant (C392S) did not impact DHE transport. Moreover, the stimulatory effect of Sac1p on DHE transport required Sac1p to be immobilized on L E liposomes. Sac1p in a soluble form did not influence DHE transport. It is thus unlikely that Sac1p works with Osh4p via direct protein–protein interactions as suggested previously [30] . In our binding assays, whatever its state (empty or in the presence of ligands), Osh4p was not recruited by Sac1p onto liposomes ( Supplementary Fig. 5b ). 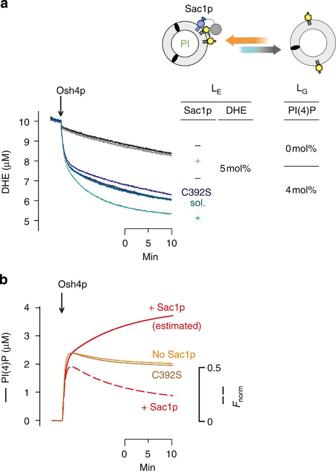Figure 3: PI(4)P hydrolysis by Sac1p on ER-like liposome sustains sterol transport by Osh4p. (a) DOPC/DOGS-NTA-Ni2+/DNS-PE/DHE liposomes (90.5/2/2.5/5 mol/mol, 200 μM total lipids, LEliposomes) were preincubated or not with Sac1p[1–522]His6or an inactive variant (C392S) and mixed with DOPC liposomes (200 μM lipids, LGliposomes) containing 0 or 4 mol% PI(4)P. After 3 min, Osh4p (200 nM) was added and DHE transport was monitored. The experiment with soluble Sac1p (200 nM) was done with LEliposomes devoid of DOGS-NTA-Ni2+. (b) The transport of PI(4)P was monitored with LEliposomes devoid of Sac1p or with LEliposomes covered by 200 nM Sac1p[1–522]His6or Sac1p[1–522]His6(C392S). The amount of PI(4)P (solid line) transported by the protein is only indicated for experiments in which no PI(4)P hydrolysis occurs. For experiments with Sac1p, only theFNormsignal is indicated (dashed line). The estimated trace corresponds to the amount of PI(4)P, which is likely transported by Osh4p into LEliposome when Sac1p is present on LEliposome and active. Figure 3: PI(4)P hydrolysis by Sac1p on ER-like liposome sustains sterol transport by Osh4p. ( a ) DOPC/DOGS-NTA-Ni 2+ /DNS-PE/DHE liposomes (90.5/2/2.5/5 mol/mol, 200 μM total lipids, L E liposomes) were preincubated or not with Sac1p[1–522]His 6 or an inactive variant (C392S) and mixed with DOPC liposomes (200 μM lipids, L G liposomes) containing 0 or 4 mol% PI(4)P. After 3 min, Osh4p (200 nM) was added and DHE transport was monitored. The experiment with soluble Sac1p (200 nM) was done with L E liposomes devoid of DOGS-NTA-Ni 2+ . ( b ) The transport of PI(4)P was monitored with L E liposomes devoid of Sac1p or with L E liposomes covered by 200 nM Sac1p[1–522]His 6 or Sac1p[1–522]His 6 (C392S). The amount of PI(4)P (solid line) transported by the protein is only indicated for experiments in which no PI(4)P hydrolysis occurs. For experiments with Sac1p, only the F Norm signal is indicated (dashed line). The estimated trace corresponds to the amount of PI(4)P, which is likely transported by Osh4p into L E liposome when Sac1p is present on L E liposome and active. Full size image In the PI(4)P transport assay, the increase in NBD-PH FAPP signal, indicative of the transfer of PI(4)P from L G to L E liposomes by Osh4p, was followed by a large decay when Sac1p was immobilized on L E liposomes ( Fig. 3b , dashed line), which was not observed with Sac1p(C392S). Undoubtedly, PI(4)P hydrolysis prevented the relocalization of NBD-PH FAPP on L E liposomes, as PH FAPP is unable to detect PI ( Supplementary Fig. 2e ), the reaction product. Thus, the NBD trace resulting from the combination of transport and hydrolysis processes was no longer a direct readout of the amount of PI(4)P transferred by Osh4p. This amount was estimated by fitting the trace with a kinetic model, (see Supplementary Methods ) which integrates the rate of PI(4)P hydrolysis by Sac1p as estimated using a distinct assay ( Supplementary Fig. 5c ). This analysis indicated that Osh4p transferred more PI(4)P ( ∼ 1.7 μM, Fig. 3b ) from L G to L E liposomes when Sac1p was attached to L E liposomes. The model used for fitting procedures seemed adequate since it fairly predicted the DHE kinetic trace in the presence of Sac1p as well as the lipid transport kinetics in the absence of Sac1p ( Supplementary Fig. 6a ). Together, these data indicated that the hydrolysis of PI(4)P by Sac1p on ER-like membranes sustains PI(4)P transport by Osh4p. In turn, this transport allows extended transport of sterol in the opposite direction. Osh4p transports sterol against its gradient by using PI(4)P To maintain a sterol gradient intracellularly, Osh4p should be able to deliver sterol from early to late membranes against its concentration gradient. Accordingly, we compared the transport of DHE by Osh4p from L E to L G liposomes in three situations: along the DHE gradient as previously measured ( Fig. 2 ), in the absence of a DHE gradient or against a DHE gradient. For this, we prepared L E liposomes containing 5 mol% DHE and L G liposomes incorporating 4 mol% PI(4)P and 0, 5 or 10 mol% DHE. In the first case, the initial DHE transport rate was similar to previous values ( ∼ 20 DHE per min per protein). Remarkably, in the second case, where DHE was already equilibrated between liposomes, we observed a very fast diminution in FRET signal on Osh4p injection, corresponding to the transfer of ∼ 1 μM DHE from L E to L G liposomes ( Fig. 4a , upper panel, dark blue trace). Moreover, in the third case, a very transient decrease was also observed, implying that Osh4p had transported DHE from L E to L G liposomes within the first seconds against its gradient. In each situation, the initial DHE transport was coupled to a backward transfer of PI(4)P of equal velocity and no DHE transport occurred if L G liposomes were devoid of PI(4)P ( Fig. 4a,b ). These observations revealed that Osh4p can create or maintain a sterol gradient between membranes owing to its sterol/PI(4)P exchange activity. 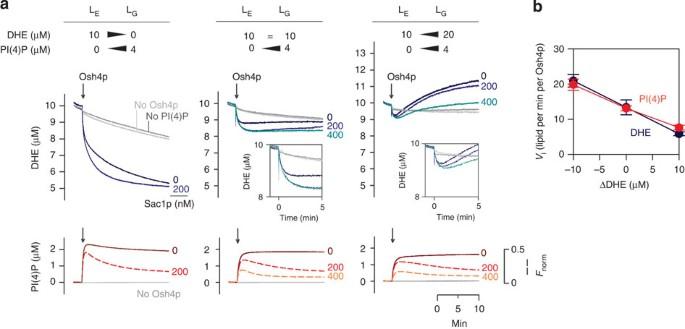Figure 4: Osh4p uses PI(4)P to create and maintain a sterol gradient. (a) Upper panel: DHE transport assay. Osh4p (200 nM) is added to DOPC/DOGS-NTA-Ni2+/DNS-PE/DHE liposomes (90.5/2/2.5/5 mol/mol, 200 μM total lipids, LEliposome) mixed with DOPC liposomes (200 μM total lipids, LGliposome) containing 0, 5 or 10 mol% DHE, with or without 4 mol% PI(4)P. Alternatively, an equivalent amount of HKM buffer was injected. Lower panel: PI(4)P transport assay. DOPC/PI(4)P/Rhod-PE liposomes (94/4/2 mol/mol, 200 μM total lipids, LGliposome) containing 0, 5 or 10 mol% DHE were incubated with NBD-PHFAPP(250 nM). Next, DOPC/DOGS-NTA-Ni2+liposomes (98/2 mol/mol, 200 μM total lipids, LEliposome) doped with 5 mol% DHE were added. PI(4)P and DHE were incorporated in the liposome at the expense of DOPC. After 3 min, Osh4p (200 nM) was injected. For experiments with Sac1p (200 or 400 nM) LEliposomes were premixed on ice for 10 min with Sac1p[1–522]His6. (b) Initial DHE and PI(4)P transport rates as a function of the difference of DHE (ΔDHE) between LGand LEliposome. The data are represented as mean±s.e.m. (error bars,n=3 for DHE transport assay andn=4 for PI(4)P transport assay) and were determined from experiments similar to that shown inaperformed in the absence of Sac1p and with LGliposome doped with 4 mol% PI(4)P. Figure 4: Osh4p uses PI(4)P to create and maintain a sterol gradient. ( a ) Upper panel: DHE transport assay. Osh4p (200 nM) is added to DOPC/DOGS-NTA-Ni 2+ /DNS-PE/DHE liposomes (90.5/2/2.5/5 mol/mol, 200 μM total lipids, L E liposome) mixed with DOPC liposomes (200 μM total lipids, L G liposome) containing 0, 5 or 10 mol% DHE, with or without 4 mol% PI(4)P. Alternatively, an equivalent amount of HKM buffer was injected. Lower panel: PI(4)P transport assay. DOPC/PI(4)P/Rhod-PE liposomes (94/4/2 mol/mol, 200 μM total lipids, L G liposome) containing 0, 5 or 10 mol% DHE were incubated with NBD-PH FAPP (250 nM). Next, DOPC/DOGS-NTA-Ni 2+ liposomes (98/2 mol/mol, 200 μM total lipids, L E liposome) doped with 5 mol% DHE were added. PI(4)P and DHE were incorporated in the liposome at the expense of DOPC. After 3 min, Osh4p (200 nM) was injected. For experiments with Sac1p (200 or 400 nM) L E liposomes were premixed on ice for 10 min with Sac1p[1–522]His 6 . ( b ) Initial DHE and PI(4)P transport rates as a function of the difference of DHE (ΔDHE) between L G and L E liposome. The data are represented as mean±s.e.m. (error bars, n =3 for DHE transport assay and n =4 for PI(4)P transport assay) and were determined from experiments similar to that shown in a performed in the absence of Sac1p and with L G liposome doped with 4 mol% PI(4)P. Full size image Initial transport rates indicated that sterol/PI(4)P exchange was slower when the pre-existing L E -to-L G sterol gradient was positive and steeper ( Fig. 4b ). The FRET signal recovery after the lipid exchange step also suggested that DHE was transferred back from L E to L G liposomes along its gradient by a PI(4)P-independent slow re-equilibration process. Simulations indicated that the shape of sterol and PI(4)P kinetic traces are primarily influenced by the direction (positive or negative) and steepness of the pre-existing DHE gradient ( Supplementary Fig. 6b ). The attachment of Sac1p on L E liposomes improved the transfer of DHE by Osh4p in all conditions ( Fig. 4a , upper panel, blue and cyan traces). Decay of the NBD signal in PI(4)P-transport assays was indicative of Sac1p hydrolysis activity ( Fig. 4a , lower panel). Moreover, a higher density of Sac1p (400 nM) on L E liposomes was required to help Osh4p operate against a steep DHE gradient, suggesting that an elevated PI(4)P consumption was necessary in that case ( Fig. 4a , cyan trace). We conclude that the maintenance of a PI(4)P gradient helps Osh4p to create and maintain a sterol gradient between membranes. Saturated lipids help Osh4p to maintain a sterol gradient The existence of a cellular sterol gradient possibly relies on the sequestration of sterol in the trans -Golgi and PM at the expense of the ER [5] due to its higher affinity for saturated glycerophospholipids and sphingolipids [1] , [31] . This process might help the delivery of sterol by Osh4p in late membranes. We tested this hypothesis by comparing the transport of DHE by Osh4p against its gradient from L E liposomes made of diunsaturated lipid (DOPC (1,2-dioleoyl- sn -glycero-3-phosphocholine), 5 mol% DHE) to L G liposomes (including 10 mol% DHE and 4 mol% PI(4)P) made either of DOPC (as before, Fig. 4 ), of monounsaturated lipid (POPC (1-palmitoyl-2-oleoyl- sn -glycero-3-phosphocholine)) or of an equal amount of DOPC and saturated sphingomyelin (SM). As shown in the Fig. 5a , the final amount of DHE transferred by Osh4p into L G liposomes was higher when the acyl-chain saturation level of these liposomes was superior to that of L E liposomes (dark blue traces). Sterol seems trapped in L G liposomes: no return of DHE from L G to L E liposomes was observed. We noted that, at the end of the kinetic with SM-containing L G liposomes, 8 μM sterol remain in L E liposomes, indicating that they are in equilibrium with an accessible pool of 8 μM in L G liposomes. Given the amount of transported sterol, this indicated that of 22 μM total sterol, 8 μM remained accessible, whereas 14 μM (63%) were shielded by SM. However, DHE did not accumulate in L G liposomes devoid of PI(4)P, demonstrating that the delivery of sterol was primarily conditioned by its exchange with PI(4)P and not its affinity for saturated lipids. 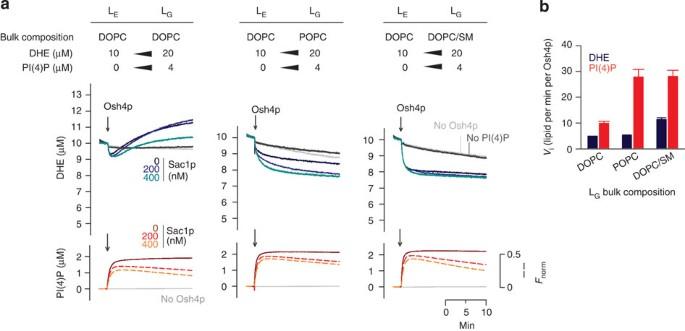Figure 5: Acyl-chain saturation in Golgi-like membranes favours sterol transport up its gradient by Osh4p. (a) Upper panel: DHE transport assay. DOPC/DOGS-NTA-Ni2+/DNS-PE/DHE liposomes (90.5/2/2.5/5 mol/mol, 200 μM total lipids, LEliposome) were mixed with DOPC/DHE (90/10 mol/mol), POPC/DHE (90/10) or DOPC/SM/DHE (45/45/10) liposomes (200 μM total lipids, LGliposome) doped, or not, with 4 mol% PI(4)P (at the expense of DOPC or POPC). Thereafter, Osh4p (200 nM) or an equivalent volume of HKM buffer was injected. Lower panel: PI(4)P transport assay. DOPC/DHE (90/10 mol/mol), POPC/DHE (90/10) or DOPC/SM/DHE (45/45/10) liposomes (200 μM lipids, LGliposome) containing 2 mol% Rhod-PE and 4 mol% PI(4)P (at the expense of DOPC) were incubated with NBD-PHFAPP(250 nM) and mixed with DOPC/DHE/DOGS-NTA-Ni2+liposomes (93/5/2 mol/mol, 200 μM lipids, LEliposome). After 3 min, Osh4p (200 nM) was added. For experiments with Sac1p, LEliposomes were premixed on ice for 10 min with Sac1p[1–522]His6. (b) Initial DHE and PI(4)P transport rates as a function of the bulk composition of LGliposomes. The data, represented as mean±s.e.m. (error bars,n=3 for DHE transport assay andn=4 for PI(4)P transport assay), were determined from experiments, as shown ina, carried out in the absence of Sac1p with LGliposomes doped with 4 mol% PI(4)P. Figure 5: Acyl-chain saturation in Golgi-like membranes favours sterol transport up its gradient by Osh4p. ( a ) Upper panel: DHE transport assay. DOPC/DOGS-NTA-Ni 2+ /DNS-PE/DHE liposomes (90.5/2/2.5/5 mol/mol, 200 μM total lipids, L E liposome) were mixed with DOPC/DHE (90/10 mol/mol), POPC/DHE (90/10) or DOPC/SM/DHE (45/45/10) liposomes (200 μM total lipids, L G liposome) doped, or not, with 4 mol% PI(4)P (at the expense of DOPC or POPC). Thereafter, Osh4p (200 nM) or an equivalent volume of HKM buffer was injected. Lower panel: PI(4)P transport assay. DOPC/DHE (90/10 mol/mol), POPC/DHE (90/10) or DOPC/SM/DHE (45/45/10) liposomes (200 μM lipids, L G liposome) containing 2 mol% Rhod-PE and 4 mol% PI(4)P (at the expense of DOPC) were incubated with NBD-PH FAPP (250 nM) and mixed with DOPC/DHE/DOGS-NTA-Ni 2+ liposomes (93/5/2 mol/mol, 200 μM lipids, L E liposome). After 3 min, Osh4p (200 nM) was added. For experiments with Sac1p, L E liposomes were premixed on ice for 10 min with Sac1p[1–522]His 6 . ( b ) Initial DHE and PI(4)P transport rates as a function of the bulk composition of L G liposomes. The data, represented as mean±s.e.m. (error bars, n =3 for DHE transport assay and n =4 for PI(4)P transport assay), were determined from experiments, as shown in a , carried out in the absence of Sac1p with L G liposomes doped with 4 mol% PI(4)P. Full size image The initial transport rate was up to three times higher with POPC or SM-containing L G liposomes, suggesting that the sterol/PI(4)P exchange was facilitated ( Fig. 5b ). Concomitantly, the transfer of DHE by Osh4p seemed moderately influenced by PI(4)P hydrolysis. A low density of Sac1p on L E liposome (200 nM) was sufficient to sustain the delivery of DHE into L G liposomes made of POPC and Sac1p became almost dispensable with SM-containing L G liposomes. We thus conclude that the higher affinity of sterol for saturated lipids [1] is a factor that facilitates Osh4p-mediated delivery of sterol against its gradient into acceptor membranes. Lipid packing defects control sterol/PI(4)P exchange The ER membrane is neutral, mostly made of unsaturated phospholipids [3] and forms extensive tubules characterized by a positive curvature [32] . Due to its unsaturation level and shape, the ER displays lipid packing defects. Such defects are known to facilitate sterol desorption as measured by in vitro assays [33] . Consequently, we examined whether the extraction of sterol by Osh4p, which should occur according to our model ( Fig. 1 ) when Osh4p is in a PI(4)P-bound form, was influenced by these defects. Osh4p[PI(4)P] was incubated with large L E liposomes made of DOPC or POPC and containing 0.5 or 5 mol% DHE (lower and upper sterol concentration in the ER [2] ). By measuring the quenching of tryptophan residues localized near the sterol-binding pocket by DHE [17] , we found that Osh4p[PI(4)P] extracted DHE from DOPC liposomes faster than from POPC liposomes ( Fig. 6a ). In each case the extraction process was accelerated when liposomes contained 5 mol% DHE. We also observed that Osh4p extracted more efficiently DHE from POPC liposomes of decreasing radius, that is, of increasing curvature ( Fig. 6b ). Eventually, we found that Osh4p in an empty state extracts more easily DHE from DOPC than POPC liposomes ( Supplementary Fig. 7a ). Thus, Osh4p efficiently exchanges PI(4)P for sterol on neutral membranes displaying lipid packing defects and containing sterol concentration similar to that found at the ER. The propensity of sterol to be extracted is likely the limiting factor of this process. 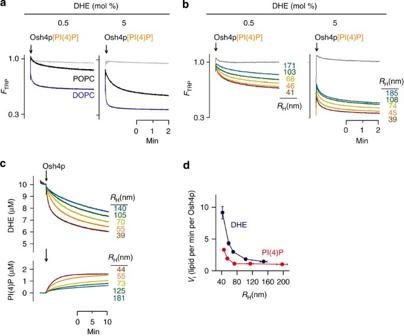Figure 6: Effect of lipid packing and curvature of LEliposomes on sterol/PI(4)P exchange. (a) Intrinsic fluorescence at 340 nm of Osh4p[PI(4)P] (500 nM) on addition to large liposomes (500 μM total lipids) made of DOPC (blue trace) or POPC (black trace), and containing 0.5 or 5 mol% DHE. A reference signal was measured with DHE-free liposomes (grey trace). (b) Osh4p[PI(4)P] (500 nM) was added to large POPC of defined radius and doped with 0.5 or 5 mol% DHE. (c) Upper panel: the transport of DHE mediated by Osh4p (200 nM) was measured between POPC/DNS-PE/DHE liposomes (92.5/2.5/5 mol/mol, 200 μM lipids, LEliposome) of defined radii and large DOPC liposomes (200 μM lipids, LGliposome) doped with 4 mol% PI(4)P. Lower panel: the transport of PI(4)P by Osh4p (200 nM) was measured with NBD-PHFAPP(250 nM) from DOPC/PI(4)P/Rhod-PE liposomes (94/4/2 mol/mol, 200 μM lipids, LGliposome) to POPC liposomes (200 μM lipids, LEliposome) of defined radius doped with 5 mol% DHE. (d) Initial transport rate for DHE and PI(4)P as deduced from the experiment shown incand plotted as a function of the hydrodynamic radius (RH) of LEliposomes. Data are represented as mean±s.e.m. (error bars,n=2). Figure 6: Effect of lipid packing and curvature of L E liposomes on sterol/PI(4)P exchange. ( a ) Intrinsic fluorescence at 340 nm of Osh4p[PI(4)P] (500 nM) on addition to large liposomes (500 μM total lipids) made of DOPC (blue trace) or POPC (black trace), and containing 0.5 or 5 mol% DHE. A reference signal was measured with DHE-free liposomes (grey trace). ( b ) Osh4p[PI(4)P] (500 nM) was added to large POPC of defined radius and doped with 0.5 or 5 mol% DHE. ( c ) Upper panel: the transport of DHE mediated by Osh4p (200 nM) was measured between POPC/DNS-PE/DHE liposomes (92.5/2.5/5 mol/mol, 200 μM lipids, L E liposome) of defined radii and large DOPC liposomes (200 μM lipids, L G liposome) doped with 4 mol% PI(4)P. Lower panel: the transport of PI(4)P by Osh4p (200 nM) was measured with NBD-PH FAPP (250 nM) from DOPC/PI(4)P/Rhod-PE liposomes (94/4/2 mol/mol, 200 μM lipids, L G liposome) to POPC liposomes (200 μM lipids, L E liposome) of defined radius doped with 5 mol% DHE. ( d ) Initial transport rate for DHE and PI(4)P as deduced from the experiment shown in c and plotted as a function of the hydrodynamic radius ( R H ) of L E liposomes. Data are represented as mean±s.e.m. (error bars, n =2). Full size image We further examined whether the membrane curvature influenced the sterol/PI(4)P exchange activity of Osh4p between L E liposomes made of POPC (with 5 mol% DHE) of defined radii and L G liposomes made of DOPC (with 4 mol% PI(4)P). With large L E liposomes ( R >100 nm), the initial transport rates were up to twentyfold lower (1.8±0.1 DHE per min and 1.1±0.3 PI(4)P per min per Osh4p ( n =2–3)) than with large L E liposomes made of DOPC ( Fig. 2 ). With POPC liposomes of decreasing radius (down to ∼ 40 nm), the velocities were partially restored ( Fig. 6c,d ). We also tested whether Osh4p can transport DHE against its concentration gradient from L E liposomes made of POPC to L G liposomes made of DOPC or POPC. Almost no transport of DHE was seen and the transport of PI(4)P in the opposite direction was also blocked ( Supplementary Fig. 7b,c ). Jointly, these data suggest that the ER constitutes a permissive membrane for sterol extraction by Osh4p in the context of sterol/PI(4)P exchange cycles because of its high curvature and its abundance in unsaturated lipids. The lid controls lipid release into neutral membranes To better apprehend the sterol/PI(4)P exchange mechanism, we examined how the binding of each lipid to Osh4p affects its structural and dynamical properties by running molecular dynamics (MD) simulations of the protein bound to ergosterol (PDB ID: 1ZHZ) or PI(4)P (3SPW). These simulations indicated that van der Waals interactions account almost exclusively (98%, Fig. 7a ) for the protein–ergosterol binding energy (216±9 kJ mol −1 ). Sterol in its binding pocket is very stable, showing little deviations from its conformation in the crystal ( Fig. 7b ). The F42, Q96 and Y97 residues contribute the most to the Osh4p–sterol interaction ( Fig. 7c ). However, each residue only participates to ∼ 7% of the total protein–sterol energy, indicating that the interaction of sterol with Osh4p relies on multiple residues. For PI(4)P, the role of electrostatic interactions was predominant, accounting for 73% of the total lipid–protein interaction energy (971±86 kJ mol −1 , Fig. 7a ). Remarkably, the PI(4)P acyl chains, despite occupying the sterol-binding pocket, showed a high flexibility compared with ergosterol ( Fig. 7b ). In contrast, the polar head of PI(4)P binds tightly to five residues (K109, H143, H144, K336 and R344; Fig. 7b,c ), which together contribute for 65% of the total PI(4)P-protein interaction energy. 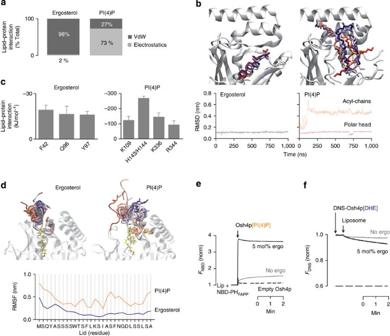Figure 7: Differential control of ligand release by the N-terminal lid of Osh4p. (a) Electrostatic and van der Waals contribution in the binding of ergosterol or PI(4)P to Osh4p. (b) Dynamic behaviour of ergosterol (left) and PI(4)P (right) inside the binding pocket of Osh4p. The time evolution of the lipids is shown during 1 μs of MD simulations with colours going from red (beginning of the MD trajectory) to blue (end of the trajectory). The root-mean-square deviation (RMSD) of ergosterol or PI(4)P polar head and acyl chains is represented. (c) Contribution to the ligand–protein interaction energy of residues that closely interact with sterol or PI(4)P. Data are represented as mean±s.d. (errors bars,n=500 time steps) (d) Motion of the N-terminal lid (residues 1–29) during 1 μs MD simulation of Osh4p bound to ergosterol (left) or PI(4)P (right). The time evolution of the lid is shown with colours going from red to blue. Lipids are shown in licorice representation. RMSF of residues 1–29 are plotted for the simulation of Osh4p bound to ergosterol (blue) or PI(4)P (orange) in the bottom panel. (e) Osh4p (500 nM) preloaded with PI(4)P was added, in the presence of NBD-PHFAPP(250 nM), to DOPC liposomes containing or not 5 mol% DHE at 30 °C. As a control, we incubated empty Osh4p. (f) DNS-Osh4p loaded with DHE (∼500 nM) was incubated at 30 °C in buffer. At the indicated time, large liposomes (with or without 5 mol% ergosterol) were injected (500 μM final lipid concentration). The release of DHE was followed by measuring the diminution in FRET between DHE and DNS-Osh4p. Figure 7: Differential control of ligand release by the N-terminal lid of Osh4p. ( a ) Electrostatic and van der Waals contribution in the binding of ergosterol or PI(4)P to Osh4p. ( b ) Dynamic behaviour of ergosterol (left) and PI(4)P (right) inside the binding pocket of Osh4p. The time evolution of the lipids is shown during 1 μs of MD simulations with colours going from red (beginning of the MD trajectory) to blue (end of the trajectory). The root-mean-square deviation (RMSD) of ergosterol or PI(4)P polar head and acyl chains is represented. ( c ) Contribution to the ligand–protein interaction energy of residues that closely interact with sterol or PI(4)P. Data are represented as mean±s.d. (errors bars, n =500 time steps) ( d ) Motion of the N-terminal lid (residues 1–29) during 1 μs MD simulation of Osh4p bound to ergosterol (left) or PI(4)P (right). The time evolution of the lid is shown with colours going from red to blue. Lipids are shown in licorice representation. RMSF of residues 1–29 are plotted for the simulation of Osh4p bound to ergosterol (blue) or PI(4)P (orange) in the bottom panel. ( e ) Osh4p (500 nM) preloaded with PI(4)P was added, in the presence of NBD-PH FAPP (250 nM), to DOPC liposomes containing or not 5 mol% DHE at 30 °C. As a control, we incubated empty Osh4p. ( f ) DNS-Osh4p loaded with DHE ( ∼ 500 nM) was incubated at 30 °C in buffer. At the indicated time, large liposomes (with or without 5 mol% ergosterol) were injected (500 μM final lipid concentration). The release of DHE was followed by measuring the diminution in FRET between DHE and DNS-Osh4p. Full size image The remarkable difference in dynamics between sterol and the PI(4)P acyl chains in Osh4p is intimately linked to the behaviour of the N-terminal lid. Stable van der Waals interactions between ergosterol and hydrophobic residues restrain lid movement. In contrast, the lid in PI(4)P-bound Osh4p is extremely mobile ( Fig. 7d ). This prompted us to examine whether Osh4p liberates more readily PI(4)P than sterol. For this aim, we monitored the kinetics of PI(4)P delivery from Osh4p, preloaded with this lipid to DOPC liposome using NBD-PH FAPP as a reporter. When the liposomes were devoid of ergosterol, we observed a slow increase in the NBD signal ( Fig. 7e , grey trace). Contrastingly with liposomes containing 5 mol% ergosterol, the NBD signal reached a plateau within seconds, suggesting that PI(4)P was quickly delivered to membranes by exchange with sterol ( Fig. 7e , black trace). Quantification of PI(4)P by the PH FAPP domain indicated that all Osh4p protein had released PI(4)P. Under identical conditions, but with a different assay [17] , we found that Osh4p, loaded with DHE, exchanged it with ergosterol very slowly (1/ t 1/2 ∼ 0.0004, s −1 , Fig. 7f ), suggesting that the lid does not readily open when covering sterol. Thus, Osh4p is more prone to deliver PI(4)P than sterol into neutral, ER-like membranes. Identifying the mechanisms that generate lipid gradients between organelles is an important issue in cell biology. By measuring a lipid exchange process with an unprecedented accuracy, we reveal that an intracellular LTP can create a lipid gradient by dissipating a PI(4)P gradient. We demonstrate that Osh4p is far more efficient when it acts as a lipid exchanger than as a mere lipid transporter. In our assays in which sterol (5 mol%) and PI(4)P (4 mol%) are in distinct membranes, Osh4p transports the two lipids along opposite routes with equivalent velocities ( ∼ 20 lipids per min), whereas lipid transport is tenfold slower when one of these two lipids is absent. Furthermore, impairing the affinity of Osh4p for either sterol or PI(4)P systematically reduces both DHE and PI(4)P transport rates. Cellular observations provide results that corroborate the sterol/PI(4)P exchange model. Under conditions where sterol is already equilibrated between membranes, Osh4p mediates the accumulation of sterol in one membrane at the expense of the other by sterol/PI(4)P exchange. Moreover, Osh4p even transports sterol against a concentration gradient, alike the gradient at the ER/Golgi interface (≤5 mol% in ER [2] , 10 mol% in trans -Golgi [15] ). The lipid exchange rates are lower ( ∼ 13 and ∼ 6 lipids per min); nevertheless, they remain comparable to the rates measured for other LTPs (STARD4: 7 sterols per min (ref. 34 ); CERT: 4 ceramides per min (ref. 35 )). This suggests that Osh4p is a genuine carrier that can create and maintain sterol gradients within cells. Our kinetic analysis indicates that Osh4p rapidly transports sterol by lipid exchange until it has fully dissipated a pre-existing PI(4)P gradient between membranes. In cells, PI(4)P gradients are maintained over time as PI(4)P is continually synthesized on late membranes and hydrolysed by Sac1p on the ER [20] , [21] , [22] , [23] . In vitro, the sterol/PI(4)P exchange activity of Osh4p is sustained in conditions where Sac1p, by hydrolysing PI(4)P, maintains the PI(4)P gradient. The final amount of sterol delivered by Osh4p against a sterol gradient is higher in membranes rich in saturated lipids, likely because sterol is sequestered in these membranes, due to a higher affinity for such lipids [1] . However, the delivery process per se remains strictly PI(4)P dependent. Conversely, the sterol extraction step of the sterol/PI(4)P cycle is facilitated by the unsaturation level and positive curvature of membranes. The ER, both highly tubulated and rich in unsaturated lipid, likely constitutes a permissive membrane for Osh4p to load sterol. Future work will be necessary to examine how lipid packing influences the propensity of PI(4)P to be extracted and released by Osh4p and how the ability of Osh4p to respond to lipid packing with its ALPS motif [36] influences its capacity to create sterol gradient. Nevertheless, our present results suggest that the difference in lipid packing at the ER/Golgi interface defines an ideal context for PI(4)P-mediated vectorial transfer of sterol by Osh4p. Given its natural abundance (32.10 3 copies per cell) [37] and its sterol transport rate driven by PI(4)P (up to 10 sterols per min per protein, against a sterol gradient), Osh4p could supply the trans -Golgi with 32.10 4 sterol molecules per min, which would next be conveyed to the PM by exocytosis. Thus, during asymmetric division, a process that lasts 2 h, Osh4p could deliver up to 60% of 60 × 10 6 sterol molecules that are necessary, along with other lipids, for doubling the PM surface of the mother cell [11] . However, the contribution of Osh4p is possibly more partial since fast bidirectional sterol fluxes exist between the ER and the PM (36 × 10 5 molecules per min) [11] and might also promote the accumulation of sterol in the PM during cell growth. Nevertheless, the ability of Osh4p to rapidly exchange sterol for PI(4)P would explain why its specific knock down influences sterol levels and its transversal distribution in the Golgi and the PM [26] , [27] , [38] and, as the release of sterol uses PI(4)P, a key lipid for post -Golgi vesicle formation [39] , why it acts as a repressor of exocytosis [40] . Several mutants such as Osh4p H143A/H144A, which do not recognize PI(4)P, have no sterol/PI(4)P exchange activity in vitro . Interestingly, they do not rescue Osh-depleted strains whose PM lack sterols and, in contrast to Osh4p WT, they are not lethal in Sec14p-deficient strains displaying limited Golgi PI(4)P levels [19] . Therefore, we propose that these mutants cannot exchange sterol for PI(4)P at the Golgi, a conclusion that is corroborated by our experiments showing the lack of effect of the H143A/H144A mutant in an heterologue system. Other mutants (Q96A, Y97F) in which a residue in close contact with sterol has been modified, still extract DHE and operate sterol/PI(4)P exchange. Furthermore, we showed that Osh4p Y97F, like Osh4p WT, displaces sterol and PI(4)P in cells. These observations are in apparent contradiction with previous studies, suggesting that the Y97F mutant is deficient in binding cholesterol [19] , [41] . However, given that DHE is, unlike cholesterol, a perfect mimetic of ergosterol, and that MD simulations and other reports [42] , [43] suggest that the interaction between Osh4p and sterol relies on numerous other residues, we conclude that the Y97 residues makes a minor contribution to sterol binding. Overall, our results better explain why Osh4p WT and the Y97F mutant behave similarly in many in vivo assays [40] , [44] and indicate that the Y97F mutant is not a loss-of-function mutant. Eventually we observed that the lid is crucial for the activity of Osh4p and, moreover, prevents the release of sterol but not PI(4)P into neutral membranes owing to its versatile dynamic. Together with previous results suggesting that the opening of the lid, when Osh4p is bound to sterol, is fast when the membrane is anionic [17] , these experiments suggest that the lid contributes to the directionality of sterol transport. The lid would not prevent Osh4p to release sterol, against its concentration gradient, into the trans -Golgi but slow down the back transport of sterol in the ER, as observed in our assays mimicking the ER/Golgi interface ( Fig. 4 ). The ability to create a lipid gradient by using PI(4)P is likely shared by other ORP/Osh proteins. Recent reports suggest that all members of this family bind PI(4)P [18] , [45] , [46] and indicate that some of them recognize a second lipid that is not sterol [47] . Therefore, a general and appealing hypothesis is that ORP/Osh proteins use PI(4)P gradients to actively convey sterol or other lipids from early to late membranes. For such mechanisms to occur, the PIP turnover should be robust enough. At steady state, PI(4)P levels are low in yeast (80,000 PI(4)P molecules per cell) [24] . This value is, however, not indicative of the amount of PI(4)P, which is hydrolysed and regenerated over time. Further cellular studies with high temporal and spatial resolution are necessary to define the interplay between PI(4)P metabolism and ORP/Osh-mediated lipid movements. Protein expression and purification Full-length Osh4p and Osh4p[30–434] were cloned in pGEX-4T-3 vector to code for glutathione S -transferase (GST)-fused constructs. The different site-specific mutations in Osh4p (Q96A, Y97F, K109A, H143A/H144A, K336E,…) were obtained by the Quikchange kit (Stratagene). The PH domain (FAPP1[1–100] construct, PH FAPP ) of the phosphatidylinositol-4-phosphate adaptor protein-1 (FAPP1) was cloned in a pGEX-4T-3 vector. A linker of nine residues was inserted by the Quikchange kit between the thrombine cleavage site and the first residue of the PH domain (NGNLSSLSA) to guarantee accessibility to thrombin. The PH FAPP sequence was next mutated to replace two solvent-accessible cysteines by serine (mutation C37S and C94S) and to introduce a cysteine into a membrane-inserting wedge of the domain (T13C). A Sac1p[1–552] fragment was PCR amplified from a initial plasmid using primers incorporating a Nhe1 and Not1 restriction site and inserted into a pET-21b(+) vector to code for a soluble form of Sac1p tagged with a C-terminal hexahistidine sequence. A single mutation was introduced to obtain a catalytically dead Sac1p (mutation C392S). All sequences of Osh4p, PH FAPP and Sac1p were checked by DNA sequencing. GST–Osh4p, GST–Osh4p[30–434] and Sac1p[1–522]His 6 were expressed in Escherichia coli at 30 °C overnight, whereas the GST–PH FAPP was expressed at 37 °C for 3 h on induction with 1 mM IPTG (at an optical density (OD) equal to 0.6 at λ =600 nm). For GST-tagged proteins, all purification steps were conducted in 50 mM Tris, pH 7.4, 120 mM NaCl and 2 mM DTT. For His 6 -tagged proteins a buffer containing 50 mM Tris, pH 7.5, 300 mM NaCl and 20 mM imidazole was used. All buffers were supplemented during the first purification steps with phenylmethanesulfonylfluoride (PMSF) (1 mM), bestatine (1 μM), pepstatine (10 μM), phosphoramidon (10 μM) and protease inhibitor tablets (Roche). Cells were lysed by a French press and the lysate was centrifuged at 200,000 g for 1 h. For GST-fused protein (Osh4p and PH FAPP ), the supernatant was applied to Glutathione Sepharose 4B beads. After three washing steps, the beads were incubated with thrombin at 4 °C overnight to cleave the GST fusion and allow the release of Osh4p or PH FAPP . All constructs contain an N-terminal GS sequence from the thrombin cleavage site. All Osh4p constructs were next purified by gel filtration on a Sephacryl S300 HR XK16–70 column. For His 6 -tagged proteins (Sac1p), the supernatant was mixed with NTA-Ni 2+ agarose beads (Qiagen). After three washing steps, proteins were eluted from the beads with buffer containing first 250 mM, then 500 mM imidazole. All Sac1p constructs were subsequently purified by gel filtration on a Sephacryl S300 HR XK16–70 column. For NBD labelling of PH FAPP , the crude eluate was mixed (after DTT removal by gel filtration on illustra NAP-10 columns (GE Healthcare)) with a 10-fold excess of N,N′-dimethyl-N-(iodoacetyl)-N′-(7-nitrobenz-2-oxa-1,3-diazol-4-yl)ethylenediamine (IANBD-amide, Molecular Probes). After 90 min on ice, the reaction was stopped by adding a 10-fold excess of L-cysteine over the probe. The free probe was removed by gel filtration on a Sephacryl S200 HR XK16–70 column. The labelled protein was analysed by SDS–PAGE and ultraviolet–visible spectroscopy. The gel was directly visualized in a fluorescence imaging system (FUJI LAS-3000 fluorescence imaging system) to detect NBD-labelled PH FAPP excited in near-ultraviolet and then stained with Sypro Orange to determine the purity of NBD-PH FAPP . The labelling yield (≈100%) was estimated from the ratio of the OD of tyrosine and tryptophan at 280 nm ( ɛ =29,450 M −1 cm −1 ) and NBD at 495 nm ( ɛ =25,000 M −1 cm −1 according to the manufacturer). The production and purification of DNS-Osh4p have been described previously [17] . For all purified proteins, the concentration was determined by a Bradford assay, by SDS–PAGE analysis using a bovine serum albumin standard curve and ultraviolet spectrometry. Lipids DOPC, POPC, liver PI, brain PI(4)P, DNS-PE, NBD-PE (1,2-dioleoyl- sn -glycero-3-phosphoethanolamine-N-(7-nitro-2-1,3-benzoxadiazol-4-yl)), Rhod-PE, DOGS-NTA-Ni 2+ and 18:0 SM (N-stearoyl-D-erythro-sphingosylphosphorylcholine or C18:0 sphingomyelin) were purchased from Avanti Polar Lipids. Ergosterol and DHE were from Sigma Aldrich. The concentration of DHE in stock solution in methanol was determined by ultraviolet spectroscopy using an extinction coefficient of 13,000 M −1 cm −1 . The preparation of radiolabelled [ 32 P]PI(4)P was described previously [17] . Liposomes preparation Lipids in stock solutions in CHCl 3 were mixed at the desired molar ratio and the solvent was removed in a rotary evaporator. For lipid films including PI(4)P or DOGS-NTA-Ni 2+ , the mix was pre-warmed to 33 °C for 5 min prior to drying under vacuum. For formulations containing [ 32 P]PI(4)P, the mixture was dried in a haemolysis tube under argon. The films were hydrated in 50 mM Hepes pH 7.2 and 120 mM K-acetate (HK buffer) to obtain a suspension of multilamellar liposomes. Alternatively, to produce liposomes loaded with sucrose, films were hydrated with 50 mM Hepes, pH 7.2, 220 mM sucrose. After five thawing–freezing cycles with liquid nitrogen, the suspensions were extruded through polycarbonate filters of 0.2-μm pore size using a mini-extruder (Avanti Polar Lipids). The extruder was set with a heating/holder block to extrude at 45 °C liposomes containing SM. To produce liposomes of defined curvature, the liposomes were extruded sequentially through 0.4, 0.2, 0.1, 0.05 and 0.03 μm (pore size) filters. The liposome hydrodynamic radius ( R H ) was estimated by dynamic light scattering in a Dyna Pro instrument. Liposomes were stored at 4 °C and in the dark when containing light-sensitive lipids (DHE, DNS-PE, ergosterol, NBD-PE and Rhod-PE) and used within 2 days. Fluorimetric activity assays All fluorimetric activity assays were carried out in a Shimadzu RF 5301-PC fluorimeter. The sample (volume 600 μl) was placed in a cylindrical quartz cell, continuously stirred with a small magnetic bar and thermostated at 30 °C. At the indicated time, sample was injected from stock solutions through a guide in the cover of the fluorimeter adapted to Hamilton syringes, such as to not interrupt the fluorescence recording. DHE transport assay A suspension (570 μl) of L G liposomes (200 μM total lipids) was incubated at 30 °C under constant stirring in HKM (HK+1 mM MgCl 2 ) buffer. After 1 min, 30 μl of L E liposomes (200 μM total lipid, final concentration) containing 2.5 mol% of DNS-PE and 5 mol% of DHE was added. The volumic concentration of DHE was equal to 10 μM. DHE is quickly equilibrated between the inner and outer leaflet of liposomes ( t 1/2 of transbilayer movement <1 min [33] ) implying that the entire DHE pool is accessible to Osh4p. After 3 min, Osh4p was injected at 200 nM. Lipid transport was followed by measuring the dansyl signal at 525 nm (bandwidth 10 nm) on DHE excitation at 310 nm (bandwidth 1.5 nm). The amount of DHE (in μM) transferred from L E to L G liposomes corresponds to 10 × (( F − F 0 )/( F max − F 0 )). F max is the signal before Osh4p injection and F 0 is the signal measured with liposomes containing 2.5 mol% DNS-PE but devoid of DHE. PI(4)P transport assay A suspension (570 μl) of L G liposome (200 μM total lipids) containing 2 mol% Rhod-PE and 4 mol% PI(4)P was incubated with 250 nM NBD-PH FAPP at 30 °C in HKM buffer under constant stirring. The volume concentration of accessible PI(4)P (in the outer leaflet) is 4 μM. After 1 min, 30 μl of L E liposome (200 μM total lipids, final concentration) were injected. After additional 3 min, Osh4p (200 nM) was injected. PI(4)P transport was followed by measuring the NBD signal at 530 nm (bandwidth 10 nm) on excitation at 460 nm (bandwidth 1.5 nm). The NBD signal mirrors the distribution of NBD-PH FAPP between L E and L G liposome. In the case of a transport process without PI(4)P hydrolysis, we could directly determine the amount of PI(4)P transported by Osh4p by normalizing the NBD signal. To do so, we measured the NBD signal ( F eq ) that corresponds to a situation, where PI(4)P is fully equilibrated between liposomes. NBD-PH FAPP (250 nM) was mixed with L E and L G liposome (200 μM total lipid each) with a size and lipid composition similar to that of the liposomes used in the transport assay, except that each contains initially 2 mol% PI(4)P. Liposome-binding assays indicated that NBD-PH FAPP is completely bound to membrane for a surface-accessible amount of PI(4)P between 2 and 4 μM ( Supplementary Fig. 2e ). Consequently, the fraction of PI(4)P on L E liposome, PI(4)P E /PI(4)P T, is directly equal to the fraction of PH FAPP on L E liposome and correspond to F Norm =0.5 × ( F − F G / F eq − F G ) with F G corresponding to the NBD signal prior to the addition of Osh4p. The amount of PI(4)P (in μM) transferred from L G to L E liposome corresponds to 4 × F Norm . Considering the amount of NBD-PH FAPP and of accessible PI(4)P in our assays, only 6.25% of PI(4)P are bound to the probe during a kinetic. Considering the maximal membrane surface that could be occupied by one PH domain (≈4.8 nm 2 , estimated from refs 29 , 48 and the total liposomes surface (L E +L G ; 5.1 × 10 16 nm 2 with an area per lipid of 0.7 nm 2 ), only 0.9% of the liposomes surface is covered by the probe. Thus it is unlikely that the ability of Osh4p to transport PI(4)P is affected by the presence of NBD-PH FAPP . PI(4)P hydrolysis assay DOPC/PI(4)P/Rhod-PE liposomes (96/2/2 mol/mol, 200 μM total lipids) and DOPC/PI(4)P/DOGS-Ni-NTA 2+ liposomes (96/2/2 mol/mol, 200 μM total lipids) were mixed with NBD-PH FAPP (250 nM) at 30 °C under constant stirring. At the indicated time, Sac1p[1–522]His 6 or Sac1p[1–522](C392S)His 6 (200 or 400 nM) was injected. The NBD signal was measured at 530 nm (bandwidth 10 nm) on excitation at 460 nm (bandwidth 1.5 nm). To calculate the amount of PI(4)P hydrolysed by Sac1p on L E liposome ( x ), we considered that the normalized NBD signal F Norm =0.5 × ( F − F G / F max − F G ) is equal to (PI(4)P E − x )/(PI(4)P T − x ) with F max corresponding to the initial signal measured prior to the injection of Sac1p and F 0 is the signal measured with NBD-PH FAPP in the presence of Rhod-PE-containing liposomes only. Considering that PI(4)P E =2 μM and PI(4)P T =4 μM at the beginning of the experiment, x is equal to (2–4 F Norm )/(1− F Norm ). DHE loading assay The loading of Osh4p with DHE is measured by following the quenching of the intrinsic fluorescence of the protein. The sample initially contained liposomes doped with 0.5 or 5 mol% DHE (500 μM total lipids) in HKM buffer and is thermostated at 30 °C under continual stirring. After 1 min, Osh4p (500 nM final concentration) was injected, from a stock solution, into the sample and its fluorescence was measured at 340 nm (bandwidth 5 nm) on excitation at 286 nm (bandwidth 1.5 nm). PI(4)P and DHE delivery assays We prepare Osh4p in complex with PI(4)P and DNS-Osh4p in complex with DHE as described previously [17] . For PI(4)P delivery, we added Osh4p-PI(4)P to large liposomes (500 μM total lipids) in the presence of 250 nM NBD-PH FAPP . PI(4)P delivery was monitored at 530 nm (bandwidth 10 nm) on excitation at 460 nm (bandwidth 1.5 nm). For DHE delivery, we added 30 μl of liposomes (stock solution 5 mM, final concentration 500 μM) to DNS-Osh4p-DHE ( ∼ 500 nM). Sterol delivery was monitored at 510 nm (bandwidth 20 nm) on excitation at 310 nm (bandwidth 1.5 nm) at 30 °C. The recordings were corrected for the light scattering signal and the dilution effect induced by liposome addition. DHE extraction assay The sample (150 μl) containing DOPC liposomes (150 μM total lipids) doped with 2.5 mol% of DNS-PE and 2 mol% of DHE was incubated at 30 °C in a small quartz cuvette. Lipid extraction was followed by recording the dansyl signal at 525 nm (bandwidth 10 nm) on DHE excitation at 310 nm (bandwidth 1.5 nm) before and 5 min after the addition of 3 μM Osh4p or mutants. The signal corresponds to F max and F , respectively; the intensity signal corresponding to the maximal DHE extraction ( F 0 ), was determined with 2 mM methyl-β-cyclodextrin. The percentage of DHE extraction is given by 100 × (1−(( F − F 0 )/( F max − F 0 )). PI(4)P extraction assay Sucrose-loaded liposomes (500 μM total lipids) containing 0.4 mol% Rhod-PE, 2 mol% PI(4)P and doped with [ 32 P]PI(4)P were mixed with Osh4p or mutants (5 μM) for 20 min at room temperature. The sample was centrifuged at 400,000 g for 20 min at 20 °C in a fixed-angle rotor (TLA 100.1). The supernatant (150 μl) was recovered and the liposome pellet, which could be easily visualized owing to the presence of Rhod-PE, was resuspended in 150 μl HKM. Both samples (supernatant and pellet) were mixed with 2 ml scintillant and counted to calculate the fraction of extracted PI(4)P. Flotation experiments Proteins (750 nM) were incubated with NBD-PE containing liposomes (750 μM total lipids) in 150 μl HKM buffer at room temperature for 5 min. The suspension was adjusted to 30% sucrose by mixing 100 μl of a 75% (w/v) sucrose solution in HKM buffer and overlaid with 200 μl HKM containing 25% (w/v) sucrose and 50 μl sucrose-free HKM. The sample was centrifuged at 240,000 g in a swing rotor (TLS 55 Beckmann) for 1 h. The bottom (250 μl), middle (150 μl) and top (100 μl) fractions were collected. The top fractions were analysed by SDS–PAGE using Sypro-Orange staining and a FUJI LAS-3000 fluorescence imaging system. Cell microinjection and imaging Purified Osh4p WT, Y97F, H143A/H144A and [30–434] mutants were dialyzed in Slide-A-Lyzer MINI Dialysis Units (Pierce) against 10 mM HEPES (pH 6.9), 140 mM KCl (microinjection solution). Cytosolic microinjections in HeLa cells (Human Cervical Adenocarcinoma cell line) plated on ibiTreat μ-Slides 4 well (Ibidi) were performed using borosilicate glass capillaries (Harvard Instrument) and a motorized micromanipulator coupled to a Femtojet pressure supplyer (Eppendorf). The microinjection solution was supplemented with 0.5 mg ml −1 AlexaFluor-conjugated 10,000 MW dextran (Molecular probes) and indicated protein at a final concentration of 100 μM. Directly following microinjection, cells were incubated with DHE in complex with MCD (1:5 ratio) for 1 min at 37 °C and washed three times in PBS. Cells were further incubated in growth medium (DMEM supplemented with 10% foetal calf serum) for 1 h before imaging. Wide-field microscopy imaging was carried out using a Leica DMIRBE microscope equipped with an Andor iXon3 blue-optimized EMCCD camera driven by Solis software (Andor). DHE was imaged using Semrock BrightLine fluorescence filters (320/40 nm bandpass filter, 347 nm dichroic beamsplitter and 390/40 nm bandpass filter). Images were acquired using a Leica HCX APO × 100/1.3 oil U-V-I objective. Images were corrected for background and analysed with a low intensity threshold or a high intensity threshold with ImageJ to respectively define the total area of the cells labelled with DHE and the bright perinuclear Golgi region. A ratio between the integrated fluorescence of each area was calculated to determine the fraction of DHE in the Golgi area. For trans -Golgi labelling, cells were fixed and immunolabelled (1:400) with sheep anti-human TGN46 polyclonal antibody (AbD Serotec, AHP500G) and a donkey anti-sheep AlexaFluor 594-conjugated secondary antibody (1:400, Invitrogen, A11016). The PI(4)P probe (OSBP PH domain with GFP at the N terminus) was cloned in a pEGFP-C1 vector. HeLa cells were transfected with lipofectamine 2000 reagent (Invitrogen) for 18 h before microinjection of purified Osh4p or related mutants. Fluorescence mean intensities of the PI(4)P probe in perinuclear and cytosol regions were measured in ImageJ. Molecular dynamics simulations All simulations are based on the crystal structure of Osh4p bound to ergosterol (PDB ID: 1ZHZ) [19] and to PI(4)P (PDB ID: 3SPW) [17] . Missing residues (notably residues 1–12 of the N-terminal lid) were added to the PI(4)P-bound structure using MODELLER9v10 (ref. 49 ). The model with the lowest DOPE score [50] was retained. All ionizable side chains, as well as the C- and N-termini were modelled in their default ionization state, with the exception of H143 and H144 residues in the PI(4)P simulations, where the two histidines were modelled as protonated to balance the negative charge of the PI(4)P molecule. The system was immersed in a box of water of ∼ 83 × 76 × 96 Å 3 containing 16,350 molecules. The box dimensions are chosen in such a way that the minimum distance between periodic images of the protein is always >25 Å during the simulation. Neutrality of the system at physiological ion concentration (120 mM) was obtained by adding 47 sodium and 37 chloride ions to the aqueous phase. The total number of atoms in our models is about 56,000. After insertion of the protein, the system was minimized using a steepest descent algorithm and then heated up to 300 K in 1,200 ps, while keeping positional restraints on crystallographic Cα atoms (Cαs) that were slowly removed in two successive runs of 3 ns at 300 K. Positional restraints on crystallographic Cαs were set to 1,000 and 100 kJ mol −1 nm −2 . The all-atom CHARMM27 (ref. 51 ) force field was used in combination with the TIP3P [52] model for water. The force field for non-standard residue ergosterol was taken from ref. 53 , while the force field for PI(4)P was adapted from ref. 54 . Electrostatic interactions were calculated with the Ewald particle mesh method [55] with a real space cutoff of 10 Å. Bonds involving hydrogen atoms were constrained using the LINCS algorithm [56] and the integration time step was set to 2 fs. The system was coupled to a Bussi thermostat [57] and to an isotropic Parrinello–Rahman barostat [57] at a temperature of 300 K and a pressure of 1 atm. The MD trajectories described in the text are the following: two MD runs of 1 μs each for Osh4p bound to PI(4)P; one MD run of 1 μs of Osh4 bound to ergosterol. All data analysis were done using GROMACS [58] utilities and all molecular images were made with Visual Molecular Dynamics (VMD) [59] . All analyses reported are performed over the last 500 ns of the trajectories; for PI(4)P the data are averaged over two independent trajectories. How to cite this article: Moser von Filseck, J. et al. A phosphatidylinositol-4-phosphate powered exchange mechanism to create a lipid gradient between membranes. Nat. Commun. 6:6671 doi: 10.1038/ncomms7671 (2015).